Sub-micron phase coexistence in small-molecule organic thin films revealed by infrared nano-imaging Controlling the domain size and degree of crystallization in organic films is highly important for electronic applications such as organic photovoltaics, but suitable nanoscale mapping is very difficult. Here we apply infrared-spectroscopic nano-imaging to directly determine the local crystallinity of organic thin films with 20-nm resolution. We find that state-of-the-art pentacene films (grown on SiO 2 at elevated temperature) are structurally not homogeneous but exhibit two interpenetrating phases at sub-micrometre scale, documented by a shifted vibrational resonance. We observe bulk-phase nucleation of distinct ellipsoidal shape within the dominant pentacene thin-film phase and also further growth during storage. A faint topographical contrast as well as X-ray analysis corroborates our interpretation. As bulk-phase nucleation obstructs carrier percolation paths within the thin-film phase, hitherto uncontrolled structural inhomogeneity might have caused conflicting reports about pentacene carrier mobility. Infrared-spectroscopic nano-imaging of nanoscale polymorphism should have many applications ranging from organic nanocomposites to geologic minerals. Highly ordered organic materials hold high promise for novel electronics [1] , [2] , [3] , [4] . Reproducible device performance rests on understanding the effect of molecular arrangement on charge-carrier mobility. Pentacene is one of the most characterized and best-performing materials for organic thin-film devices [2] , [5] , [6] . To maximize its mobility, the most crucial parameters for pentacene quality have been identified to be the substrate and its temperature during deposition [1] , [5] , [6] , [7] . On the one hand, substrate temperatures well above 50 °C result in larger grains of the film structure with characteristic lengths of microns [8] . On the other hand, deposition temperature also controls the abundance of several crystallographic phases, such as thin-film phase (TFP) and bulk phase (BP) pentacene [5] , [6] , [9] . Here we reveal the surprising lateral nanostructure of two coexisting pentacene polymorphs on a 300-nm scale, by mapping infrared absorption using a near-field infrared microscope [10] . We observe ellipse-shaped BP pentacene ubiquitously within the dominant TFP, uncorrelated with grain structure. Our finding may explain why the carrier mobility ceases to increase in pentacene thin films deposited at elevated substrate temperature despite increased grain size [5] , [11] , [12] ; apparently, BP nucleation obstructs charge transport by scattering off polarons from inter-phase boundaries [1] , [13] . Furthermore, we observe that the BP pentacene grows over months at room temperature without a change of grain morphology, as we also corroborate by X-ray diffraction. The BP ellipses come with a subtle topographical depression, which earlier had led to interpretation of them as cracks [14] , [15] . Infrared nanoscopy clearly has a high potential for analyzing the molecular arrangement of organic thin films at the nanoscale and thus for better understanding organic electronic systems. X-ray diffraction shows recrystallization during storage The crystallographic phases in pentacene films can be discriminated by their (001)-spacing of the molecular layers. For the TFP, the pentacene molecules are oriented almost perpendicularly on the substrate and the (001)-spacing amounts to 15.4 Å, while for the BP it is 14.4 Å [9] , [16] , [17] as the molecules are slightly tilted, shown in the inset of Fig. 1 . The sample studied in Fig. 1 was grown at 65 °C to obtain large crystalline grains. After deposition, X-ray diffraction measurements showed that the film was dominated by TFP, with some weak fraction of BP ( Fig. 1 , yellow curve) as expected for deposition temperatures above 50 °C [5] , [18] . However, surprisingly, the BP fraction was found considerably increased at the expense of TFP (red curve) after the sample had been stored over 20 months in a desiccator at room temperature (23 °C). This observation by itself is an alarming signal for pentacene-based device development and calls for immediate attention. 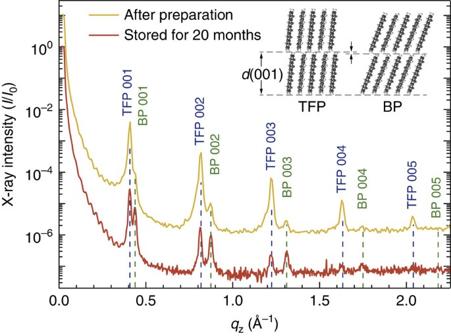Figure 1: Recrystallization in highly ordered pentacene film. X-ray diffraction of a 40-nm thick pentacene layer acquired right after fabrication (yellow curve), and after storage at room temperature for 20 months (red curve, vertically offset). The blue and green dashed lines indicate the positions of the (00L) Bragg peaks due to TFP and BP pentacene, respectively, corresponding to their well-known (001)-spacings of 15.4 and 14.4 Å (refs5,9). Aging decreases TFP peaks and increases BP peaks. This observation clearly indicates a recrystallization from TFP to BP within the pentacene film. The two different molecular arrangements for TFP and BP, as well as their layer spacingd(001) perpendicular to the substrate are depicted in the inset. Figure 1: Recrystallization in highly ordered pentacene film. X-ray diffraction of a 40-nm thick pentacene layer acquired right after fabrication (yellow curve), and after storage at room temperature for 20 months (red curve, vertically offset). The blue and green dashed lines indicate the positions of the (00 L ) Bragg peaks due to TFP and BP pentacene, respectively, corresponding to their well-known (001)-spacings of 15.4 and 14.4 Å (refs 5 , 9 ). Aging decreases TFP peaks and increases BP peaks. This observation clearly indicates a recrystallization from TFP to BP within the pentacene film. The two different molecular arrangements for TFP and BP, as well as their layer spacing d (001) perpendicular to the substrate are depicted in the inset. Full size image Infrared nano-imaging reveals elliptic BP inclusions As the X-ray experiment geometry does not provide lateral information, additional methods are needed to determine the domain geometries and to understand how the phase conversion takes place in detail. An atomic force microscopy (AFM) image of the stored sample is shown in Fig. 2a . The film exhibits a grainy structure on the expected characteristic lateral length scale of 2–5 μm [6] . On the one hand, there is the argument that larger grains are beneficial for high charge-carrier mobility, simply as any kind of grain boundary will naturally impose a barrier due to defects, lowering the mobility [6] , [7] , [13] . On the other hand, film deposition at increased substrate temperatures to obtain large grains led to diverging results of increased [1] , almost unchanged [11] , and even reduced [5] carrier mobility. In addition, even for pentacene films deposited at constant substrate temperature, the mobility tends to saturate with increasing grain size [12] , [19] . In a similar direction, Shtein et al . [20] have reported that in some cases smaller grains allow for higher mobility, while others observed that post-annealing reduces mobility due to structure variation and nucleation of BP pentacene [21] , [22] . Unfortunately in the experimental studies, it remains unclear whether apparent individual grains as observed by AFM are single crystals, and in particular, whether and on what scale BP and TFP domains are arranged. Thus, resolving the lateral crystallinity and the organization of BP and TFP pentacene might resolve the conflicting reports on the interplay between growth temperature, apparent grain size and charge transport in pentacene films. 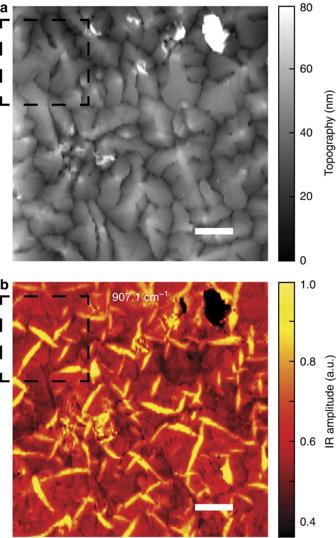Figure 2: Grain morphology and lateral distribution of two coexisting phases. (a) AFM topography (13.5 μm × 13.5 μm) showing a 40-nm thick pentacene film on SiO2/Si substrate, after storage at room temperature for 20 months. (b) s-SNOM amplitude image at 907.1 cm−1, recorded simultaneously, proves the coexistence of two phases of pentacene, which obviously persist across grain boundaries. The dashed square marks the section shown inFig. 4. Scale bar, 2 μm. Figure 2: Grain morphology and lateral distribution of two coexisting phases. ( a ) AFM topography (13.5 μm × 13.5 μm) showing a 40-nm thick pentacene film on SiO 2 /Si substrate, after storage at room temperature for 20 months. ( b ) s-SNOM amplitude image at 907.1 cm −1 , recorded simultaneously, proves the coexistence of two phases of pentacene, which obviously persist across grain boundaries. The dashed square marks the section shown in Fig. 4 . Scale bar, 2 μm. Full size image To map and contrast BP and TFP domains in pentacene thin-film devices, we employ scattering-type scanning near-field optical microscopy (s-SNOM) with mid-infrared illumination, as it is known from far-field measurements that the different packing of TFP and BP pentacene results in a small shift of infrared vibrational frequencies [23] , [24] , [25] . s-SNOM enhances AFM probing by an additional channel of local infrared spectroscopy and should allow imaging the local distribution of both phases with a lateral resolution given by the probing tip diameter of typically 20 nm (see Methods) [10] . The near-field infrared image of the stored pentacene film shown in Fig. 2b was recorded using mid-infrared illumination at 907.1 cm −1 , which is close to the resonance of BP pentacene [23] . Strikingly, the infrared map is not homogeneous at all but exhibits ubiquitous nanoscale features, at strong contrast, in the form of bright and highly elongated ellipsoids, which, according to the choice of the infrared frequency, originate from BP domains. These domains appear uncorrelated to the topographic morphology recorded simultaneously ( Fig. 2a ), as they even persist across grain boundaries. Many BP ellipsoids are oriented approximately perpendicularly with respect to their neighbours and appear to stay mutually aligned within larger domains comprising several grains. Crystalline packing of molecules shifts local infrared resonance To investigate the spectral origin of this strong infrared contrast, we employ a fully spectroscopic mode of the s-SNOM, recently termed nano-FTIR (nanoscale Fourier transform infrared spectroscopy) [26] , [27] that registers broad near-field spectra at each sample position, here one on a BP ellipsoid and one on TFP next to it ( Fig. 3 , as marked in the left inset). A Lorentzian fit to each spectrum confirms the two distinctly different vibrational resonances on the BP ellipsoid, peaked at 906 cm −1 (green curve), and on the surrounding TFP, peaked at 904 cm −1 (blue curve). These frequencies agree well with literature values of TFP and BP pentacene [23] , [24] . A vertical, dashed line in the spectra of Fig. 3 indicates the specific frequency used for monochromatic imaging in Fig. 2b (907.1 cm −1 , CO 2 laser line P08). At this frequency, the nano-FTIR absorption on the BP ellipsoid (green curve, Fig. 3 ) is more than twice as high compared with the surrounding TFP material (blue curve), explaining the bright contrast observed in Fig. 2b . 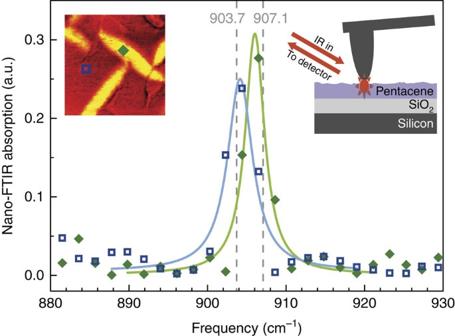Figure 3: Structural phases can be distinguished by an infrared resonance shift. Nano-FTIR spectra (data points) of a 40-nm thick pentacene film on SiO2/Si substrate taken at two different positions that are marked in the left inset, taken fromFig. 4b(on ellipsoid—green and off ellipsoid—blue). For each spectrum, 20 interferograms with 5 min acquisition time each were averaged. We chose to record 4.8-mm long interferograms to attain 2.1 cm−1spectral resolution (interferometer configuration as in ref.26,Fig. 1). As seen from the Lorentzian fits (curves) to the data, the spectrum taken on the BP ellipsoid (green curve) clearly shows a higher resonance frequency (906 cm−1) than that of surrounding TFP (904 cm−1, blue curve). The CO2laser lines (P08, P12) used for monochromatic imaging (Figs 2and4) are indicated by vertical dashed lines. The right inset sketches the principle of back-scattering SNOM. Figure 3: Structural phases can be distinguished by an infrared resonance shift. Nano-FTIR spectra (data points) of a 40-nm thick pentacene film on SiO 2 /Si substrate taken at two different positions that are marked in the left inset, taken from Fig. 4b (on ellipsoid—green and off ellipsoid—blue). For each spectrum, 20 interferograms with 5 min acquisition time each were averaged. We chose to record 4.8-mm long interferograms to attain 2.1 cm −1 spectral resolution (interferometer configuration as in ref. 26 , Fig. 1 ). As seen from the Lorentzian fits (curves) to the data, the spectrum taken on the BP ellipsoid (green curve) clearly shows a higher resonance frequency (906 cm −1 ) than that of surrounding TFP (904 cm −1 , blue curve). The CO 2 laser lines (P08, P12) used for monochromatic imaging ( Figs 2 and 4 ) are indicated by vertical dashed lines. The right inset sketches the principle of back-scattering SNOM. Full size image For a final verification of the optical response of the BP features observed in Fig. 2b , we applied the monochromatic imaging mode of the s-SNOM to a smaller sample area, with both the previous ( Fig. 4a–c ) and a slightly shifted illumination frequency ( Fig. 4e,f ). As expected, changing from 907.1 cm −1 to 903.7 cm −1 , near the TFP resonance [23] , [24] , results in a reversion of the infrared amplitude contrast ( cf . Fig. 4e ). This invertible contrast proves that (i) infrared s-SNOM can selectively highlight either BP or TFP pentacene simply by choice of the infrared frequency, and that (ii) BP and TFP domains coexist on a ca . 300-nm length scale and seem to be not at all correlated to the well-known grain structure. This experimental finding is very surprising, as it allows us to conjecture that BP pentacene nucleates in the form of nanometre inclusions within, rather than on top of, TFP pentacene. BP seeds seem hidden in the morphology of the TFP and grow with storage time, as indicated by our X-ray analysis above ( Fig. 1 ). In addition, s-SNOM imaging of a thick pentacene film (120 nm average thickness) shows that pentacene BP aggregates forming on top of the thick film [18] act as growth seeds for BP nucleation throughout the film underneath (see Supplementary Fig. 1 ). The strong infrared contrasts of our s-SNOM images appear homogeneous within BP ellipses as well as among ellipses. As the probing depth of s-SNOM is of the order of the tip diameter [10] , here 20–30 nm, the observed homogeneity suggests that BP material in the ellipses is not mixed with TFP and extends through the full film depth. 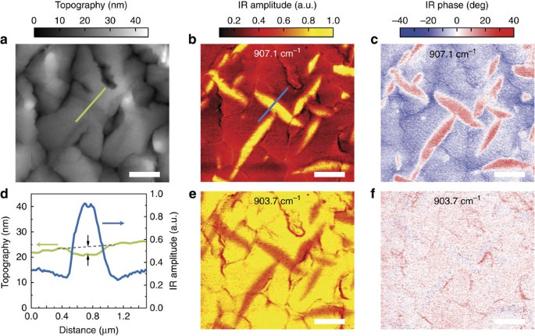Figure 4: Infrared contrast and topographic depression confirm BP nucleation. Two s-SNOM measurements (monochromatic imaging mode) of the same section of the pentacene film (5 μm × 4.5 μm) marked by the dashed square inFig. 2. The two repeats were conducted at different infrared illumination frequencies of 907.1 cm−1(a–c) and 903.7 cm−1(e,f), corresponding to the CO2laser lines P08 and P12, respectively. Characteristic BP pentacene ellipsoids appear both in the infrared amplitude (b,e) and phase (c,f) images. Clearly, changing the illumination frequency inverts the relative contrast between pentacene polymorphs in both the amplitude and phase images. Line profiles across a BP domain (d) illustrate a subtle depression in topography (green curve) marked with arrows, and a strong contrast in the infrared amplitude (blue curve). Scale bar, 1 μm. Figure 4: Infrared contrast and topographic depression confirm BP nucleation. Two s-SNOM measurements (monochromatic imaging mode) of the same section of the pentacene film (5 μm × 4.5 μm) marked by the dashed square in Fig. 2 . The two repeats were conducted at different infrared illumination frequencies of 907.1 cm −1 ( a – c ) and 903.7 cm −1 ( e , f ), corresponding to the CO 2 laser lines P08 and P12, respectively. Characteristic BP pentacene ellipsoids appear both in the infrared amplitude ( b , e ) and phase ( c , f ) images. Clearly, changing the illumination frequency inverts the relative contrast between pentacene polymorphs in both the amplitude and phase images. Line profiles across a BP domain ( d ) illustrate a subtle depression in topography (green curve) marked with arrows, and a strong contrast in the infrared amplitude (blue curve). Scale bar, 1 μm. Full size image A close inspection of the AFM micrograph reveals that it is indeed possible to discern the BP ellipses also in topography, as subtle depressions of several nanometre depth ( Fig. 4a ), quantified in extracted line profiles (green curve, Fig. 4d ). A similar observation had earlier been noted in the literature [14] , [15] . There, the depressions were interpreted as cracks in the pentacene film and thought to be induced by its greater contraction compared with the substrate on cooling down to room temperature after deposition. Our experiments indeed suggest an alternative mechanism, in which the mechanical stress is relaxed by a continuous conversion of TFP into BP pentacene at the interface boundaries. The direction of this phase change is determined by BP pentacene exhibiting a larger unit-cell footprint along the substrate plane compared with TFP [16] , [28] , thus slowing the contraction and reducing the mechanical tension. In previous work, a phase transition from pentacene TFP to BP during storage under ambient air was related to the difference between the surface energies and the bulk energies of the two pentacene phases [29] , [30] . However, a theoretical study has already suggested that surface stress makes a contribution to this crystallization as well [31] . Here, the driving force is indeed the reduction of mechanical tension induced by the thermal contraction mismatch between pentacene and the substrate. Although our study focuses on pentacene on commonly used SiO 2 substrate, we expect a similar behaviour for other substrates that feature a thermal expansion coefficient different from the one of pentacene. Our observation that the BP ellipsoids appear aligned along predominant, orthogonal directions ( Fig. 2b , presumably the crystal axes of TFP) supports the conjectured evolution of BP from highly ordered TFP pentacene. The phase conversion from the initial, upright molecular orientation of TFP easily explains why the resulting BP has the molecules also upright on the substrate, as proven in X-ray diffraction by its 14.4 Å (001)-spacing ( Fig. 1 ). Indeed, this height is by 1 Å smaller than that of TFP, due to a larger tilt of the molecules ( cf . inset Fig. 1 ) [9] , [16] , [17] . As the 40-nm thick pentacene sample consists of about 30 molecular layers, the accumulated topographical depression should be ~3 nm, as is experimentally demonstrated in the AFM line profile ( Fig. 4d , green line). This agreement confirms that the nanoscale BP ellipses penetrate the full film depth. Thus, despite our well-controlled growth of pentacene films with optimized topographical homogeneity, BP ellipses may well dissect percolation pathways in TFP and hinder carrier transport, a phenomenon that has escaped discovery so far in spite of the large number of studies on this material. The influence of BP crystallization on carrier mobility might be further investigated by recording the BP evolution in the channel of a working field-effect transistor (see Supplementary Fig. 2 ) or even by direct measurements of the local conductivity via the SNOM technique [32] . During storage of the pentacene sample, BP continues to grow at the expense of TFP pentacene (see Supplementary Fig. 3 ), which may turn out to be critical for the shelf life of pentacene electronic devices. Altogether, our method of infrared contrasting at nanoscale resolution has straightforwardly clarified that the larger grains in pentacene films deposited at elevated substrate temperature (65 °C) are subject to massive nucleation of nanometre-sized BP inclusions in the dominant TFP. We expect that the unique combination of molecular specificity (which includes sensitivity to molecular arrangement) and nanometre resolution offered by the infrared near-field interaction will allow to deepen our understanding of the nanostructure of conjugated and aromatic materials for organic electronics. Our findings demonstrate that s-SNOM is ideally suited for monitoring polymorphism and phase coexistence in highly ordered organic films at 20-nm resolution. We also foresee great opportunities for infrared s-SNOM in the field of semi-crystalline polymers, where the nanometer-scale coexistence of crystalline and amorphous phases [33] , [34] with fullerene domains [35] , [36] is discussed in the context of exciton and charge transport. Imaging of the acceptor and donor network in terms of structure and composition should considerably help to better understand organic photovoltaics. Pentacene deposition The pentacene samples were prepared on Si substrate on top of 20-nm thick thermally grown SiO 2 . The Si/ SiO 2 substrates were successively cleaned by sonication in acetone and isopropyl alcohol for 10 min each, followed by thorough rinsing with deionized water and then dried with nitrogen. Molecular beam deposition was employed to prepare 40-nm thick films, using triple-sublimed pentacene (Sigma-Aldrich), at a deposition rate of 0.2 Å s −1 , a substrate temperature of 65 °C and a pressure of about 2 × 10 −6 mbar. X-ray diffraction X-ray intensity measurements were carried out by reflectometry using a laboratory X-ray diffractometer with a Mo-K α source (wavelength λ =0.71 Å). The scattered X-ray intensity was normalized and plotted against the momentum transfer q z =(4 π / λ ) sin θ , where λ is the wavelength and θ the scattering angle. s-SNOM near-field microscope We employed a commercial scattering near-field microscope (NeaSNOM, neaspec.com ) equipped with a standard metallized tip (NCPt arrow, nanoandmore.com ), operated in AFM tapping mode at 50 nm amplitude to modulate the near-field interaction between the tip and sample. The back-scattered infrared signal is detected simultaneously with the topography (see sketch in the right inset of Fig. 3 ). Lock-in and heterodyne detection at the n =3 harmonic of the tapping frequency (~300 kHz) provides background-free near-field imaging. Monitoring of the infrared signal versus tip-sample separation (approach curves) was used to ensure the optimal working settings of the tapping amplitude, the demodulation order n and the focusing. In the monochromatic infrared near-field imaging mode ( Figs 2 and 4 ) a line-tunable 13 C 16 O 2 laser attenuated to 10 mW was used for illumination. The acquisition time was 9 ms per pixel, requiring several minutes for a 300 × 300 pixel-sized image. Nano-FTIR mode of s-SNOM The spectroscopic mode of s-SNOM ( Fig. 3 ) employs illumination by a coherent broadband mid-infrared beam (here 25 μW) from a home-built difference-frequency source driven by a <100-fs Er fibre laser (FFS.SYS-2B with FFS-CONT, toptica.com ) [26] . Detection and spectral analysis of the back-scattered light is carried out via an asymmetric Michelson interferometer that generates, by online Fourier transformation, infrared amplitude and phase spectra simultaneously. Note that although common FTIR spectrometers are not equipped to determine the complete, complex material response, the nano-FTIR phase spectra valuably complement the amplitude spectra [26] , [27] . Specifically, nano-FTIR absorption by molecular vibrational resonance can be directly determined by multiplying the measured scattering amplitude with sin( ϕ ), where ϕ is the measured scattering phase [27] . The work of F. Huth, et al . [27] also demonstrates that near-field infrared spectra of organic substances, that is, weak oscillators, exhibit indeed the same spectral positions, spectral widths and relative intensities as the corresponding far-field spectra. How to cite this article: Westermeier, C. et al . Sub-micron phase coexistence in small-molecule organic thin films revealed by infrared nano-imaging. Nat. Commun. 5:4101 doi: 10.1038/ncomms5101 (2014).